Xenoturbella bockiexhibits direct development with similarities to Acoelomorpha Xenoturbella bocki , a marine animal with a simple body plan, has recently been suggested to be sister group to the Acoelomorpha, together forming the new phylum Xenacoelomorpha. The phylogenetic position of the phylum is still under debate, either as an early branching bilaterian or as a sister group to the Ambulacraria (hemichordates and echinoderms) within the deuterostomes. Although development has been described for several species of Acoelomorpha, little is known about the life cycle of Xenoturbella . Here we report the embryonic stages of Xenoturbella , and show that it is a direct developer without a feeding larval stage. This mode of development is similar to that of the acoelomorphs, supporting the newly proposed phylum Xenacoelomorpha and suggesting that the last common ancestor of the phylum might have been a direct developer. Xenoturbella bocki Westblad, 1949 is a marine worm about 1-cm long with a simple acoelomate body plan, lacking an anus, organized gonads and a brain [1] . Because of this simple organization, its phylogenetic position has long remained contentious [2] . Although recent molecular phylogenetic analyses agree that Xenoturbella is related to the Acoelomorpha, there is still controversy as to whether this clade is an early bilaterian offshoot [3] or forms a new phylum Xenacoelomorpha as a sister group to the Ambulacraria (hemichordates and echinoderms) within the deuterostomes [4] . Developmental studies that may provide data to help resolve this discrepancy have been performed on a number of acoelomorph species [5] , [6] , [7] , but until now, little has been known about the development of Xenoturbella bocki. Brooded embryos have been reported previously [8] , but DNA sequence analyses are lacking and further studies are essential to verify their identity. Brooded larvae with molluscan larval characteristics have also been reported [9] , but as the animal has been shown to prey on bivalve molluscs [10] , [11] these seem to be most parsimoniously interpreted as food items. Here we report for the first time the observation of non-brooded developmental stages of Xenoturbella . Observations on live specimens Adult Xenoturbella bocki were kept in aquarium culture and monitored for the presence of eggs. Fertilized eggs were found on two occasions. On the first, six eggs were found and collected, from which one swimming embryo hatched the following day. On the second occasion, 73 eggs were produced which, when collected, gave rise to seven swimming hatchlings and one unhatched embryo on the following day. Naturally spawned eggs sank to the bottom of the dish even after the mucus surrounding them was removed. Eggs were pale orange and opaque, with a diameter of 205±9 μm (mean±s.d., n =10) ( Fig. 1a ) and surrounded by a transparent layer with a space of 35±3 μm ( n =10). PCR on DNA extracted from three eggs and a swimming-stage embryo using primer pairs to amplify mitochondrial cytochrome c oxidase 1 ( cox1 ) produced a 715-nucleotide fragment identical in sequence to that of Xenoturbella bocki . 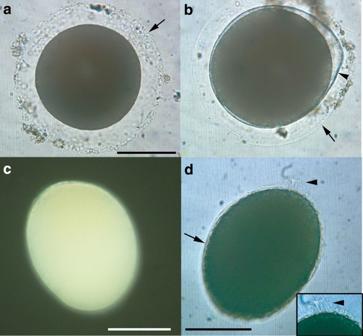Figure 1: Eggs and hatchling ofXenoturbella bocki. (a) Unfertilized egg with a transparent layer (arrow). (b) Embryo before hatching within the fertilization envelope (arrowhead), surrounded by the transparent outer layer (arrow). (c) Embryo a day after hatching with anterior end at top left. (d) Embryo 3 days after hatching, uniformly covered with cilia (arrow). Apical tuft (arrowhead) at top right, also shown enlarged in inset. Scale bars, 100 μm. Figure 1: Eggs and hatchling of Xenoturbella bocki . ( a ) Unfertilized egg with a transparent layer (arrow). ( b ) Embryo before hatching within the fertilization envelope (arrowhead), surrounded by the transparent outer layer (arrow). ( c ) Embryo a day after hatching with anterior end at top left. ( d ) Embryo 3 days after hatching, uniformly covered with cilia (arrow). Apical tuft (arrowhead) at top right, also shown enlarged in inset. Scale bars, 100 μm. Full size image The single live, unhatched embryo was found rotating within two extracellular layers. The thicker inner one, presumably the fertilization envelope, surrounded the embryo tightly within the outer layer present in unfertilized eggs ( Fig. 1b and Supplementary Movie 1 ). The newly hatched embryos were yellowish, almost spherical ( Fig. 1c ), about 209-μm long ( n =4), and swam close to the water surface with a clockwise rotation when seen from the posterior ( Supplementary Movie 2 ). Hatched embryos were reared at 4–10 °C in filtered sea water until fixation. Free-swimming stages were extremely fragile, and only limited observations were possible. At 3 days after hatching, the embryos had elongated along the anterior–posterior axis, reaching ~230 μm in length and 200 μm in width, and swam near the water surface with a rotating motion ( Supplementary Movie 3 ). Individuals were uniformly ciliated with cilia about 5- to 10-μm long, apart from an apical tuft at the anterior end with very long cilia about 20–30 μm in length ( Fig. 1d ). The apical tuft on the anterior of the animal had a rather wide base, and is in this respect different from apical tufts seen in protostome trochophore larva. No mouth or blastopore was observed. Internal morphology revealed by confocal microscopy Confocal microscopy observations of a fixed and cleared 4-day specimen revealed a fully differentiated ectoderm 40- to 80-μm thick, comprising a single layer of narrow epithelial cells, some containing glandular vesicles 2–5 μm in diameter ( Fig. 2a ). The ectoderm surrounds an internal cavity, which is outlined by a thin dark cellular layer ( Fig. 2b ). The cavity is primarily filled with round undifferentiated cells with a diameter of 17–22 μm ( Fig. 2a ). The anterior part of the cavity contained larger cells about 30 μm across ( Fig. 2c ), while the posterior part was filled with an extracellular mass containing small cells about 10 μm in diameter and round vesicles with diameters of 2–3 μm ( Fig. 2d ). No epithelial structures such as archenteron, coelomic cavities/spaces or epithelial pouches were observed ( Fig. 2e ). The absence of a mouth, vestibule, anus or archenteron shows that the Xenoturbella embryo is non-feeding and, as suggested by their opaque yolky appearance, is lecithotrophic. 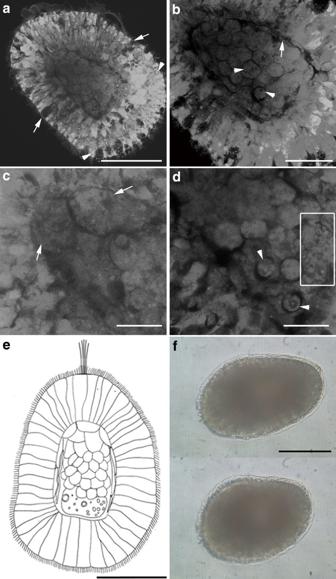Figure 2: Free-swimming stages ofXenoturbella bocki. (a–d) Confocal microscopy, 4 days after hatching with anterior at upper left. (a) Epithelial ectoderm (developing to epidermis) with glandular cells (arrows) and vesicles (arrowheads) surrounding the internal cell mass (developing to gastrodermis). (b) Thin dark layer of developing subepidermal muscle cells (arrow) surrounds the gastrodermal cell mass, composed of rounded cells. Arrowheads point to the nuclei of the rounded cells. (c) Large cells in the anterior part of the internal cavity (arrows). (d) Small cells (arrowheads) and extracellular vesicles (inside square) in the posterior part of the internal cavity. (e) Diagram of a 4-day hatchling ofXenoturbella bocki, based on the specimen ina. Anterior to top. (f) Free-swimming specimen 5 days after hatching before (upper panel) and after (lower panel) contracting the body. Anterior end at left. Scale bars, 100 μm (a,e,f); 50 μm (b); 25 μm (c,d). Figure 2: Free-swimming stages of Xenoturbella bocki . ( a – d ) Confocal microscopy, 4 days after hatching with anterior at upper left. ( a ) Epithelial ectoderm (developing to epidermis) with glandular cells (arrows) and vesicles (arrowheads) surrounding the internal cell mass (developing to gastrodermis). ( b ) Thin dark layer of developing subepidermal muscle cells (arrow) surrounds the gastrodermal cell mass, composed of rounded cells. Arrowheads point to the nuclei of the rounded cells. ( c ) Large cells in the anterior part of the internal cavity (arrows). ( d ) Small cells (arrowheads) and extracellular vesicles (inside square) in the posterior part of the internal cavity. ( e ) Diagram of a 4-day hatchling of Xenoturbella bocki , based on the specimen in a . Anterior to top. ( f ) Free-swimming specimen 5 days after hatching before (upper panel) and after (lower panel) contracting the body. Anterior end at left. Scale bars, 100 μm ( a , e , f ); 50 μm ( b ); 25 μm ( c , d ). Full size image At 5 days after hatching, the embryo became barrel-shaped, measuring 255 μm in length and 150 μm in width ( Fig. 2f ). Individuals continued to swim near the surface but occasionally glided on the bottom of the dish. At this stage, they were able to contract using internal musculature ( Fig. 2f and Supplementary Movie 4 ). No animals survived beyond this stage. Ultrastructural observations using electron microscopy Ultrastructural studies of cross-sections of a 4-day-old specimen show a well-developed epidermal layer surrounding a gastric cell mass without a cavity ( Fig. 3a ). The parenchymal cell layer that is located between the gastrodermis and the muscle sac in adults [1] has not yet formed at this stage. Rounded bodies with heterogeneous flocculent content were present in both the gastric cells and the cells of the epidermal layer, although they were more numerous in the former. They are presumed to be symbiotic bacteria ( Fig. 3a ), similar to those found in the adult [12] . The gastric cells also contain many homogeneous, round granules, possibly yolk or lipid granules. 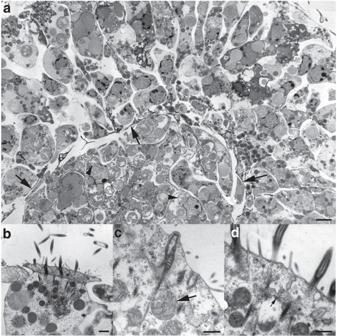Figure 3: Transmission electron microscopy of 4-day free-swimming hatchling ofXenoturbella bocki. (a) Cross-section of the body. Note the thin electron-dense cytoplasmic extensions of muscle cells, delimiting the outer epidermal layer from the inner gastrodermal cell mass (arrows). Many rounded bodies, presumed to be symbiotic bacteria, are present in the gastrodermal cells (arrowheads). Scale bar, 2 μm. (b) Surface of a multiciliated epidermal cell with ciliary axonemes and double vertical rootlets. The epidermal cells are laterally interdigitating. Scale bar, 1 μm. (c) Epidermal cell surface with double ciliary rootlets in longitudinal section. Note mitochondria (arrow) close to rootlets. Scale bar, 0.5 μm. (d) Epidermal cell surface with ciliary rootlets. Note microtubuli spreading out from the ciliary basal foot (arrow). Scale bar, 0.5 μm. Figure 3: Transmission electron microscopy of 4-day free-swimming hatchling of Xenoturbella bocki . ( a ) Cross-section of the body. Note the thin electron-dense cytoplasmic extensions of muscle cells, delimiting the outer epidermal layer from the inner gastrodermal cell mass (arrows). Many rounded bodies, presumed to be symbiotic bacteria, are present in the gastrodermal cells (arrowheads). Scale bar, 2 μm. ( b ) Surface of a multiciliated epidermal cell with ciliary axonemes and double vertical rootlets. The epidermal cells are laterally interdigitating. Scale bar, 1 μm. ( c ) Epidermal cell surface with double ciliary rootlets in longitudinal section. Note mitochondria (arrow) close to rootlets. Scale bar, 0.5 μm. ( d ) Epidermal cell surface with ciliary rootlets. Note microtubuli spreading out from the ciliary basal foot (arrow). Scale bar, 0.5 μm. Full size image The epidermal cells are laterally interdigitating, most prominently near the surface ( Fig. 3b ), as in the adult epidermis [13] . The epidermal ciliary apparatus also has a very similar substructure to that of the adult [13] , with a vertically oriented first rootlet emerging from the anterior face of the basal body, and a thicker, vertically oriented second rootlet emerging as a direct continuation of the basal body ( Fig. 3b ). Microtubules radiate from the ciliary basal foot to interconnect with other ciliary rootlet units ( Fig. 3d ). The epidermal cilia appear to have a narrow distal shaft-like structure, very similar to that present in the adult [13] . Cross-sections of the distal parts of the cilia show that they are either full size with a central doublet and nine peripheral doublets, or half size with central axonemal doublets and 4 or 5 of the peripheral doublets. None were smaller, indicating that the cilium is not evenly tapering but ends bluntly, with a distalmost shaft-like section. The microvilli dispersed among the cilia are simple and unbranched. Many rounded mitochondria can be seen close to the ciliary rootlets ( Fig. 3b–d ). Below the epidermal cells that reach the surface there are epidermal supporting cells ( Fig. 3a ), and among them also gland cells filled with mucus granules that open to the epidermal surface. The substructure and contents of these gland cells are similar to those found in the adult [13] . A developing muscle sac consisting of muscle cells with narrow and long cytoplasmic extensions ( Figs 3a and 4a ) delimits the inner gastrodermal body part from the outer epidermal layer. The muscle cells show at this stage little differentiation between the outer circular muscle layer, and the inner longitudinal layer in the adult [14] . The muscles contain myofilaments in bundles ( Fig. 4b ). The irregular myofilaments in the muscle cells are similar to what has been reported from the adult [14] . The irregularity is slightly more pronounced compared with the adult, but this is probably because the muscle cells are not fully developed. 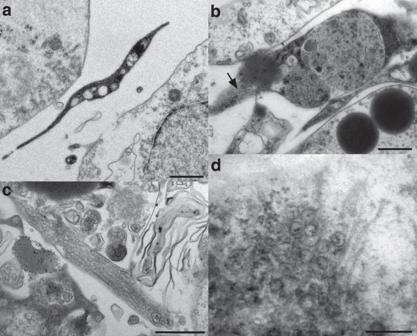Figure 4: Transmission electron microscopy of 4-day free-swimming hatchling ofXenoturbella bocki. (a) Cytoplasmic extension of developing muscle cell, situated between the epidermal cell layer and the gastric cell mass. Scale bar, 0.5 μm. (b) Developing muscle cell with electron-dense cytoplasm and myofilament bundles in cross-section, also seen in oblique section (arrow). Scale bar, 0.5 μm. (c) Part of developing muscle cell, showing myofilaments in longitudinal section. Scale bar, 0.5 μm. (d) Point-core neuronal vesicles and neurotubules in nerve cell synapse. Scale bar, 0.25 μm. Figure 4: Transmission electron microscopy of 4-day free-swimming hatchling of Xenoturbella bocki . ( a ) Cytoplasmic extension of developing muscle cell, situated between the epidermal cell layer and the gastric cell mass. Scale bar, 0.5 μm. ( b ) Developing muscle cell with electron-dense cytoplasm and myofilament bundles in cross-section, also seen in oblique section (arrow). Scale bar, 0.5 μm. ( c ) Part of developing muscle cell, showing myofilaments in longitudinal section. Scale bar, 0.5 μm. ( d ) Point-core neuronal vesicles and neurotubules in nerve cell synapse. Scale bar, 0.25 μm. Full size image A developing nerve plexus is located basiepithelially, with nerve cells containing neurotubules and vesicles at the synapses and nerve ends ( Fig. 4d ). There are few nerve cells and synapses at this stage, but they are already similar to those of the adult stage [15] . There were no visible traces of an extracellular matrix between the ectodermal epithelial layer and the muscle cell layer. This was apparently yet to develop in later stages. Many authors have emphasized the importance of Xenoturbella development for the understanding of metazoan and deuterostome evolution [2] , [8] , [9] , [10] , [15] , and the results presented here are the first report of naturally spawned eggs and free-swimming stages from Xenoturbella since the animal was described in 1949 (ref. 1 ). Both the sequence analyses and morphological observations reported here rule out that the eggs and embryos are from bivalves. The observed hatchlings swam for 5 days, and by that time their tissues had differentiated to a similar degree as in the adults [13] , [14] , [15] , including an epidermal ciliary apparatus, a muscle sac and basiepidermal nerve cells ( Figs 3 and 4 ). Some differences to the adults were found, including the absence of an extracellular matrix (that is, basal lamina) and the lack of muscle cells differentiated into circular and longitudinal muscles. Feeding structures, such as a mouth, anus, vestibule and differentiated gut, were absent at this 5-day stage. Gastric cells contained large amounts of yolk or lipids ( Fig. 3a ), a feature common in lecithotrophic marine larvae. Except for the apical tuft, the embryo showed no other visible larval-specific structural features such as larval arms, ridges or ciliary bands. Based on these observations, we conclude that Xenoturbella bocki has direct development without a feeding larva. The observed embryonic stages of Xenoturbella are similar to 3- to 4-day-old embryos of the direct-developing acoel Neochildia fusca [6] . At this stage, organogenesis in the acoel has given rise to a ciliated epithelium as well as differentiated muscle cells, both surrounding a central mass of undifferentiated gastric cells. Our observations show a similar anatomical organization in 4-day Xenoturbella embryos, with a ciliated epithelium ( Figs 2a and 3 ), a central mass of undifferentiated spherical cells ( Figs 2a , b and ) and a thin layer of developing muscles in between ( Figs 2b , 3a and 4a–c ). The latter was observed contracting 5 days after hatching ( Fig. 2f and Supplementary Movie 4 ). Recent molecular phylogenomic analyses group Xenoturbella and Acoelomorpha together in the new phylum Xenacoelomorpha [3] , [4] . A close relationship between these two groups has long been suggested based on morphology [1] , [13] , [16] , and the similarities of their developmental stages as reported in this study add further support to their sister group relationship. We suggest that the last common ancestor of Xenacoelomorpha developed through a non-feeding uniformly ciliated embryo with an undifferentiated gastric cell mass. This juvenile stage later matures into a ciliated worm with a blind gut and a simple nervous system. Two hypotheses are possible for the origin of the simple morphology found in Xenacoelomorpha direct-developing embryos. The first is that an ancestral feeding larval stage was lost entirely, and direct development was secondarily derived. A possibility that acoels stem from an ancestor with a feeding larva has recently been suggested based on neuroanatomy of an acoel [17] , supporting this view. An apical tuft is present in Xenoturbella hatchlings and some cnidarian planula larvae [18] but absent from free-swimming stage acoels [5] , [6] , [7] , suggesting that at least some secondary simplification has occurred in acoel development. There are numerous reports of echinoderm and hemichordate species that have secondarily lost a feeding-stage larva [19] , [20] , [21] , and the same may have also taken place in the Xenacoelomorpha ancestor. The second hypothesis is that the simple morphology is a plesiomorphic feature retained from the metazoan ancestor. The similarities observed in Xenacoelomorpha hatchlings, cnidarian planula larvae and poriferan parenchyma larvae support this view. As noted above, there are many marine species that have secondarily simplified a feeding larval stage, but these species usually possess vestigial ciliary bands, mouth, anus, vestibule or gut [19] , [20] , [21] , [22] , none of which were found during Xenoturbella or Acoelomorpha development. Presently, it is difficult to ascertain whether their direct development is an ancestral or a derived feature. Currently, there are conflicting views on the phylogenetic relationships of Xenacoelomorpha, some suggesting that the phylum belongs at the base of the bilaterians [3] , and others regarding them as deuterostomes [4] . The latest phylogenomic analyses suggest the latter, which has also gained support by the presence of a deuterostome-specific GNE kinase in Xenacoelomorpha [23] . Currently, the deuterostome relationship seems probable, but no planktotrophic larval stages or vestigial feeding structures have been reported from Acoelomorpha, and they were not found in Xenoturbella in this study either, offering few phylogenetically informative features to resolve this issue. If Xenacoelomorpha is an early bilaterian offshoot, it is parsimonious to regard direct development as retained from the metazoan ancestor, while a feeding larva may have been acquired in the bilaterian ancestor after Xenacoelomorpha has branched off ( Fig. 5a ). If Xenacoelomorpha is a deuterostome, Xenacoelomorpha direct development may result from the entire loss of feeding larval structures, as dipleurula larvae, seen in extant echinoderms and hemichordates, are suggested to have been present in the deuterostome ancestor [21] , [24] ( Fig. 5b ). However, it is also possible that the simple morphology of the swimming stage in Xenacoelomorpha may have been retained from the metazoan ancestor ( Fig. 5c ). This implies that feeding larvae with ciliary bands present in protostomes and deuterostomes may be the result of convergent evolution ( Fig. 5c ), which is in agreement with previous hypotheses based on morphology and gene expression [25] , [26] , [27] . Moreover, if Xenacoelomorpha is a sister taxon to the Ambulacraria [4] , it further implies that the dipleurula-type larva, which has previously been suggested to be at the origin of the chordate body plan [28] , [29] , [30] , [31] , may have arisen in the Ambulacrarian lineage after Xenacoelomorpha separated from it ( Fig. 5c ). 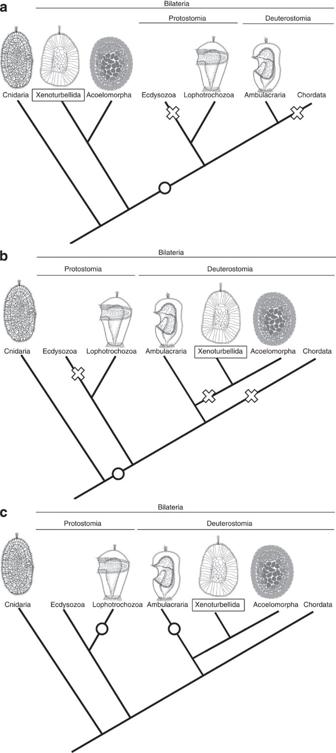Figure 5: Hypotheses on the evolution of metazoan development. Acquisition of feeding larvae shown with circles, and loss of feeding larvae shown with crosses. (a) Xenacoelomorpha as an early offshoot of the bilaterians suggested by Hejnolet al.3Similarities with cnidarian planula may indicate an ancestral developmental stage for metazoans. (b,c) Xenacoelomorpha as deuterostomes suggested by Phillipeet al.4(b) If Xenacoelomorpha direct development was secondarily derived, feeding larvae may have been lost independently in Ecdysozoa, Xenacoelomorpha and Chordata. (c) If Xenacoelomorpha direct development was retained from the metazoan ancestor, planktotrophic larvae with ciliary bands may have been independently acquired in the Ambulacraria and the Lophotrochozoa. Drawings of Acoelomorpha are modified from Ramachandraet al.6, those of Lophotrochozoa and Ambulacraria from Arendtet al.34, and Cnidaria from Kammet al.35, respectively. Figure 5: Hypotheses on the evolution of metazoan development. Acquisition of feeding larvae shown with circles, and loss of feeding larvae shown with crosses. ( a ) Xenacoelomorpha as an early offshoot of the bilaterians suggested by Hejnol et al. [3] Similarities with cnidarian planula may indicate an ancestral developmental stage for metazoans. ( b , c ) Xenacoelomorpha as deuterostomes suggested by Phillipe et al. [4] ( b ) If Xenacoelomorpha direct development was secondarily derived, feeding larvae may have been lost independently in Ecdysozoa, Xenacoelomorpha and Chordata. ( c ) If Xenacoelomorpha direct development was retained from the metazoan ancestor, planktotrophic larvae with ciliary bands may have been independently acquired in the Ambulacraria and the Lophotrochozoa. Drawings of Acoelomorpha are modified from Ramachandra et al. [6] , those of Lophotrochozoa and Ambulacraria from Arendt et al. [34] , and Cnidaria from Kamm et al. [35] , respectively. Full size image We have shown here that Xenoturbella development can, with some difficulty, be followed in the laboratory. Further studies on Xenacoelomorpha development and comparisons with cnidarian and deuterostome species are essential to determine whether its direct development is an ancestral or a derived feature. Further studies are also needed to elucidate important embryonic features that remain unidentified, such as cleavage pattern, gastrulation and mouth formation. However, modern developmental methods such as gene expression studies, immunohistochemistry and transmission electron microscopy often depend on a reasonable number of embryos, which are presently not accessible from this species. Hence, morphological and gene expression studies on adult Xenoturbella , together with genome analyses shall also prove helpful in understanding the origins and evolution of Xenoturbella . Collecting animals Adult Xenoturbella bocki were collected as previously reported in [11] . Nine animals collected on 12 January 2007 were kept in a closed 50-ml tube with filtered sea water at 4–8 °C. Fertilized eggs found in the tube after 3 days were transferred to a clean Petri dish and maintained at 4 °C. A total of 24 adults collected on 9 February 2007 were kept in mud (sieved with a 500-μm mesh) in a flask with a mesh (pore size 100 μm) placed on both the inflow and the outflow tubes. Fertilized eggs were found trapped on the outflow mesh on 28 February 2007. All eggs were transferred to Petri dishes and kept at 10 °C in filtered sea water. Pictures of eggs and embryos were taken with a Canon S40 colour camera adapted to Leica DMRBE or MZFLIII microscopes. Confocal laser scanning microscopy Embryos were fixed in 2.5% glutaraldehyde in 0.1 M sodiumcacodylate buffer (pH 7.2) for 6–16 h at 4 °C and washed with 0.1 M sodiumcacodylate buffer (pH 7.2). Fixed specimens were cleared by gradually transferring them into glycerol and observed using confocal microscopes TCS SPE (Leica) and TCS SP5 (Leica). Autofluorescence was used to observe the internal structures of the cleared animals. Transmission electron microscopy One embryo was fixed using 2.5% glutaraldehyde buffered in 0.1 M sodiumcacodylate (pH 7.2) at 5 °C for about 3 h on ice. The material was then rinsed in sodiumcacodylate buffer and postfixed in 1% osmium (buffered in 0.1 M sodiumcacodylate) at 5 °C for about 1 h, then rinsed again and stored in the buffer at 4 °C. The material was later dehydrated in an acetone/ethanol series, transferred to propyleneoxide and subsequently embedded in EPON. Sections were cut at a thickness of 1 μm, and stained with toluidine blue. Ultrathin sections (60–90 nm) were stained with uranyl acetate and lead citrate [32] . Digital micrographs were obtained with a Phillips CM 10 (Aarhus University) at magnifications between 5,000 and 46,000 using a high voltage of 60 kV and a Kodak Megaplus 1.6i Camera. All micrographs were analysed using cellSens Dimension 1.7 software (Olympus Soft Imaging Solutions GmbH, Münster, Germany). PCR and sequence analyses DNA was extracted from three naturally spawned eggs and one embryo using QIAamp DNA Micro Kit (Qiagen) following the manufacturer’s instructions. PCRs were carried out on an ABI 2720 thermal cycler using cox1 primers LCO 1490 (5′-GGTCAACAAATCATAAAGATATTGG-3′) and HCO 2198 (5′-TAAACTTCAGGGTGACCAAAAAATCA-3′) from [33] and PuReTaq Ready-To-Go PCR Beads (GE Healthcare). PCR amplification consisted of 95 °C at 3 min for 1 cycle, 95 °C at 30 s, 50 °C at 30 s and 72 °C at 1 min for 45 cycles and 72 °C at 8 min for 1 cycle. PCR products were purified using Exo-Sap (Fermentas GmbH), and sequenced with Applied Biosystems 3130xl Genetic Analyser. Sequences were analysed using 4Peaks (by A. Griekspoor and Tom Groothuis, http://mekentosj.com ) and BlastX at NCBI ( http://www.ncbi.nlm.nih.gov/blast/Blast.cgi ). The sequence for the Xenoturbella swimming stage has been deposited in GenBank under accession number JX277096. Accession codes: Sequence data have been deposited in GenBank under accession code JX277096 . How to cite this article: Nakano, H. et al. Xenoturbella bocki exhibits direct development with similarities to Acoelomorpha. Nat. Commun. 4:1537 doi: 10.1038/ncomms2556 (2013).